Observing optical coherence across Fock layers with weak-field homodyne detectors Quantum properties of optical modes are typically assessed by observing their photon statistics or the distribution of their quadratures. Both particle- and wave-like behaviours deliver important information and each may be used as a resource in quantum-enhanced technologies. Weak-field homodyne (WFH) detection provides a scheme that combines the wave- and particle-like descriptions. Here we show that it is possible to observe a wave-like property such as the optical coherence across Fock basis states in the detection statistics derived from discrete photon counting. We experimentally demonstrate these correlations using two WHF detectors on each mode of two classes of two-mode entangled states. Furthermore, we theoretically describe the response of WHF detection on a two-mode squeezed state in the context of generalized Bell inequalities. Our work demonstrates the potential of this technique as a tool for hybrid continuous/discrete-variable protocols on a phenomenon that explicitly combines both approaches. Quantum correlations play a central role in our understanding of fundamental quantum physics and represent a key resource for quantum technologies [1] , [2] , [3] , [4] . Progress in quantum information science has followed an increasingly thorough understanding of how such correlations manifest themselves and how they can be successfully generated, manipulated and characterized [5] . In quantum optical systems, these correlations appear in either properties of the fields, such as quadrature entanglement, or at the level of individual quanta, that is, photons. Access and control over such correlations are key to applications in quantum information science; however, how the complementary mode and particle correlations precisely act as a resource is still a subject of debate [6] . The capability of studying the correlations in a regime traversing mode and particle aspects is thus necessary for clarifying the origin of quantum enhancement. When a coherent superposition of many photons occupies a single mode, a wave-like description of the quantum state in terms of continuous variables (that is, the values of the quadratures) of the electromagnetic field is the standard approach [7] . The canonical technique for measuring such light fields is strong-field homodyne detection, which directly probes the quadratures of a field and can provide a full reconstruction of its quantum state [8] . On the other hand, particle-like properties can be directly accessed with a range of photodetectors, a notable example being photon-number-resolving detectors (PNRDs) [9] , [10] , [11] , [12] , and suitable techniques for the reconstruction of the photon statistics [13] , [14] . However, such photon counters are intrinsically insensitive to phase, and thus cannot access any coherence between modes. Weak-field homodyne (WFH) has been proposed as a measurement technique bridging wave- and particle-like descriptions [15] , [16] , [17] , [18] , [19] , [20] , [21] . As in standard homodyne, a local oscillator (LO) provides phase sensitivity, while the photon statistics are accessed by number-resolving detectors. The main difference is that WFH makes use of a classical reference whose mean photon number is of a similar order as that of the probed signal; this allows for the combination of the homodyne technique with PNRDs based on photon counting modules. In this paper, we employ WFH detection to investigate coherence between different photon-number basis states (Fock layers) across two-mode entangled states. Our detection scheme accesses this manifestation of optical coherence directly, without the need for resource-intensive full state tomography. We demonstrate the oscillations of an array of multi-photon coincidence counts when a split single-photon state (SSPS) and a two-mode squeezed state (TMSS) are interfered with a weak LO. Our experiment can be regarded as a first step towards the quantitative study of the nonlocal properties of multi-mode quantum states with multi-outcome measurements by non-Gaussian detectors. To this end, we theoretically study a violation of Bell inequalities that can be achieved for low numbers of detected photons under ideal conditions. Experiment The WFH setup is depicted in Fig. 1a . A signal is mixed on a beam splitter with a local oscillator, described by the coherent state | αe iφ ›, which establishes a phase reference. One or both output modes from the beam splitter are then detected using PNRDs. The method is termed ‘weak-field’ since the intensity of the LO is comparable to that of the signal. This differs from strong-field homodyne in which the coherent state is many orders of magnitude more intense than the signal, and the outputs are detected by linear photodiodes. 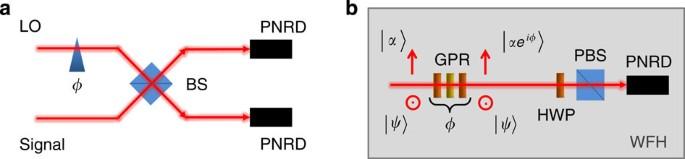Figure 1: Layout of the WFH detector. (a) The general scheme relies on the interference between a signal and a LO of similar intensity for different settings of the phaseφ. Either one or both outputs are measured with PNRDs. (b) Our experimental implementation adopts a collinear configuration in which the signaland the LO have orthogonal polarizations. For this reason, the beam splitter inais replaced by a half-wave plate (HWP) and a PBS that realize interference in polarization. The phase setting of the LO is controlled by means of a geometric phase rotator (GPR), which consists of a quarter-wave plate (QWP), a HWP and a second QWP. The rotation of the HWP (with both QWP fixed at 45°) applies a phase shift to the coherent state. A TMD records click events on the transmitted output mode. Figure 1: Layout of the WFH detector. ( a ) The general scheme relies on the interference between a signal and a LO of similar intensity for different settings of the phase φ . Either one or both outputs are measured with PNRDs. ( b ) Our experimental implementation adopts a collinear configuration in which the signal and the LO have orthogonal polarizations. For this reason, the beam splitter in a is replaced by a half-wave plate (HWP) and a PBS that realize interference in polarization. The phase setting of the LO is controlled by means of a geometric phase rotator (GPR), which consists of a quarter-wave plate (QWP), a HWP and a second QWP. The rotation of the HWP (with both QWP fixed at 45°) applies a phase shift to the coherent state. A TMD records click events on the transmitted output mode. Full size image To understand how WFH can detect coherence across Fock layers, consider the detection of m photons. These can originate from any Fock term | k › in the signal together with m − k photons from the LO; if the complex coefficients of the terms {| k ›} have well-defined relative phases, then these result in a modulation of the detection probability p ( m ) as the phase of the LO is varied. For a two-mode state, the relevant phases are the ones between joint detection events coming from terms in the signal of the form | k 1 ›| k 2 ›. Consequently, coherence across such events can be observed in the modulation of joint detection probabilities. We use the layout shown in Fig. 1b to study the coherence between Fock layers across the two modes of a split single photon and a squeezed vacuum state. To maximize the passive phase stability of our setup, we adopt a compact design in which the LO and the signal are collinear and occupy two orthogonal polarizations of a single spatial mode. Our PNRDs are time-multiplexed detectors (TMDs) that split an incoming beam into two spatial and four temporal modes, thereby resolving up to eight photons probabilistically using two avalanche photodiodes [10] , [22] . Specifically, the TMDs allow us to decompose the intensity of the interference patterns resulting from each output mode into its constituent photon components. In this way, we can probe pair-wise correlations between the individual Fock layers as we build up a joint detection statistics matrix, every row and column representing the number of clicks in each detected mode. The click statistics gives us access to higher-order Fock states ( k ≥1), although this detection scheme is not fully equivalent to a number-resolving detector [23] . A split single-photon state may be written as which describes a single photon in a coherent superposition of modes A and B (see Fig. 2a and Supplementary Fig. 1 for further details on the experimental layout). The results of our investigation for the SSPS are reported in Fig. 3 . 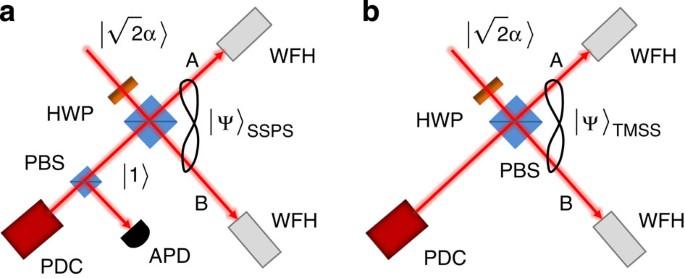Figure 2: Probing correlations across optical modes with WFH. (a) A single photon is produced by a heralded source based on parametric downconversion. We then split the single-photon state to generate |Ψ›SSPSacross two separate spatial modes (A and B), both probed by the WFH detectors described inFig. 1b. (b) The same downconversion source produces the squeezed vacuum state whose two modes are also probed by WFH detectors. Figure 2: Probing correlations across optical modes with WFH. ( a ) A single photon is produced by a heralded source based on parametric downconversion. We then split the single-photon state to generate |Ψ› SSPS across two separate spatial modes (A and B), both probed by the WFH detectors described in Fig. 1b . ( b ) The same downconversion source produces the squeezed vacuum state whose two modes are also probed by WFH detectors. 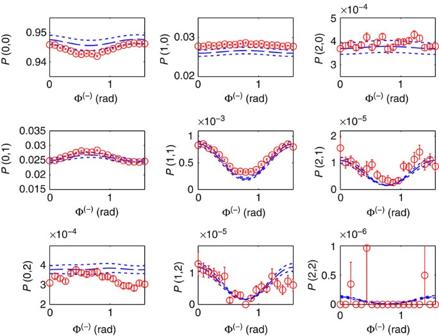Figure 3: Joint counting statistics for the SSPS. Correlations between the responses of two WFH detectors as a function of the phase difference Φ(−)=φ(−)/4 (where Φ(−)is determined by the settings of the half-wave plates in the phase rotators). We recall thatP(m,m′) is associated to the joint detection probability ofmphotons on mode A andm′ photons on mode B. The red dots are measured probabilities, with uncertainties determined by a Monte Carlo routine under the assumption of a Poissonian distribution for the raw counts. The blue theoretical curves are obtained from a model that includes the main imperfections in the setup. The dashed curves correspond to an input state with the experimentally determined weightsw0=0.161 andw1=0.669. The uncertaintiesσ0=0.011 onw0andσ1=0.029 onw1are estimated by a Monte Carlo routine; the dotted curves show the results given by the theoretical model with (w0−σ0,w1−σ1) and (w0+σ0,w1+σ1), respectively. The quantum efficiencies of the detectors,ηA=0.072 andηB=0.064, are experimentally estimated with the Klyshko method44,45. The intensities of the two local oscillators are |αA|=0.510 and |αB|=0.585. Full size image Figure 3: Joint counting statistics for the SSPS. Correlations between the responses of two WFH detectors as a function of the phase difference Φ (−) = φ (−) /4 (where Φ (−) is determined by the settings of the half-wave plates in the phase rotators). We recall that P ( m , m ′) is associated to the joint detection probability of m photons on mode A and m ′ photons on mode B. The red dots are measured probabilities, with uncertainties determined by a Monte Carlo routine under the assumption of a Poissonian distribution for the raw counts. The blue theoretical curves are obtained from a model that includes the main imperfections in the setup. The dashed curves correspond to an input state with the experimentally determined weights w 0 =0.161 and w 1 =0.669. The uncertainties σ 0 =0.011 on w 0 and σ 1 =0.029 on w 1 are estimated by a Monte Carlo routine; the dotted curves show the results given by the theoretical model with ( w 0 − σ 0 , w 1 − σ 1 ) and ( w 0 + σ 0 , w 1 + σ 1 ), respectively. The quantum efficiencies of the detectors, η A =0.072 and η B =0.064, are experimentally estimated with the Klyshko method [44] , [45] . The intensities of the two local oscillators are | α A |=0.510 and | α B |=0.585. Full size image The red dots show the experimental probabilities P ( m , m ′) of the joint detection of m clicks in mode A and m ′ clicks in mode B. Each P ( m , m ′) term is a function of the difference between the phase settings of the weak LOs, φ (−) = φ A − φ B , since a single photon has no phase per se [24] , [25] . Our count rates are such that we only consider events where m , m ′≤2; detection outcomes greater than this level are negligible. The blue lines are predictions from a model that accounts for the following imperfections in our experiment: non-unit efficiency of the detectors; modulation of the reflectivities of the beam splitters preceding the TMDs when varying the LO phases (due to the geometric phase rotators depicted in Fig. 1b —see Methods and Supplementary Fig. 2 ). We also include imperfections in the production of the single-photon states [26] , and we thus write where w 0 and w 1 are coefficients taken between 0 and 1 that weight the zero- and one-photon contributions to the input state. We experimentally determine these parameters from the photon statistics of the initial state (see Supplementary Note 1 and Supplementary Note 2 ). The experimental curves show oscillations in the coincidence counts: these are evident in the P (1, 1), P (2, 1) and P (1, 2) terms, as also predicted by the theory. What is most striking about the observed oscillatory behaviour is the fact that it is displayed by terms P ( m , m ′) for which m + m ′>1, yet it is determined by the coherence between the terms |0› A |1› B and |1› A |0› B (see equation (1)), which do not contain more than one photon each. Ideally, any additional photon detected must therefore come from the LOs, hence the SSPS is responsible for the coherent oscillations observed in the considered joint detection probabilities. In practice, we observe good qualitative agreement between the experimental data and our theoretical description. Indeed, we are able to account for all the main features of a 3-by-3 array of multi-photon counts with one model that has no free parameters; detection efficiencies and the weights in equation (2) are experimentally determined. We attribute the residual discrepancies to two main factors: imperfect mode matching between the LOs and the signal modes and variations of the laser power during the few-hour-long acquisition. An analogous experiment is conducted on a TMSS (see Fig. 2b and Supplementary Fig. 3 for further details on the experimental layout). This state is archetypal of a quantum resource with well-known correlations between its Fock layers. The expression for a TMSS reads where the real squeezing parameter λ governs the photon distribution across the photon-number basis states. Here, we pump our source with moderate parametric gain to generate significant higher-order Fock layers in the two-mode state [27] . The expected phase dependence of { P ( m , m ′)} for a TMSS was shown to be φ (+) = φ A + φ B (ref. 28 ). The TMSS has a phase dependence arising from that of the pump; in a conventional strong homodyne setup this would define which quadratures are squeezed. In our case, the same effect is manifested in the phase dependence of the click patterns; hence, appropriate phase locking was necessary (see Methods). The results obtained for the TMSS are illustrated in Fig. 4 . Once again, we observe good qualitative agreement between our data and the predictions from a theoretical model that includes the same imperfections as for the single-photon case. 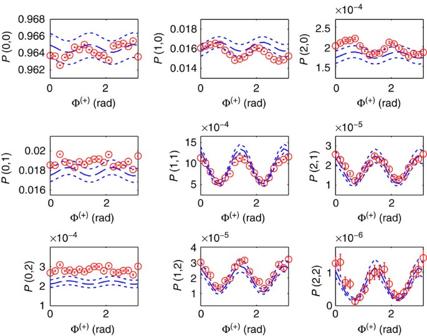Figure 4: Joint counting statistics for the TMSS. Correlations between the responses of two WFH detectors as a function of the phase sum Φ(+)=φ(+)/4 (where Φ(+)is determined by the settings of the half-wave plates in the phase rotators). We recall thatP(m,m′) is associated to the joint detection probability ofmphotons on mode A andm′ photons on mode B. The red dots are measured probabilities, with uncertainties determined by a Monte Carlo routine under the assumption of a Poissonian distribution for the raw counts. The blue theoretical curves are obtained from a model that includes the main imperfections in the setup. The dashed curves correspond to an input state with the experimentally determined squeezing parameterλ=0.295 and weightP=0.04 for the additional noise term. The uncertaintyσ=0.016 onλis estimated by a Monte Carlo routine; the dotted curves show the results given by the theoretical model withλ±σ. The experimental quantum efficiencies of the detectors areηA=0.132 andηB=0.155 (estimated with the Klyshko method). The intensities of the two local oscillators are |αA|=0.365 and |αB|=0.347. Here the input state can be modelled as Figure 4: Joint counting statistics for the TMSS. Correlations between the responses of two WFH detectors as a function of the phase sum Φ (+) = φ (+) /4 (where Φ (+) is determined by the settings of the half-wave plates in the phase rotators). We recall that P ( m , m ′) is associated to the joint detection probability of m photons on mode A and m ′ photons on mode B. The red dots are measured probabilities, with uncertainties determined by a Monte Carlo routine under the assumption of a Poissonian distribution for the raw counts. The blue theoretical curves are obtained from a model that includes the main imperfections in the setup. The dashed curves correspond to an input state with the experimentally determined squeezing parameter λ =0.295 and weight P =0.04 for the additional noise term. The uncertainty σ =0.016 on λ is estimated by a Monte Carlo routine; the dotted curves show the results given by the theoretical model with λ ± σ . The experimental quantum efficiencies of the detectors are η A =0.132 and η B =0.155 (estimated with the Klyshko method). The intensities of the two local oscillators are | α A |=0.365 and | α B |=0.347. Full size image where the extra term is a first-order approximation of noise in a squeezed thermal state. This asymmetry across the modes is justified by the experimentally recorded g (2) for the parametric downconversion source: we find and for the two marginals, to be compared with g (2) =2 for an ideal thermal state. The lower value of motivates the addition of the noise term on output mode B. The quoted values of g (2) also suggest that additional (and undesired) Schmidt modes might be responsible for the presence of photons in modes correlated to undetected modes [29] . As for the case of the SSPS, imperfect mode matching between the LOs and the signal modes and variations of the laser power during the data acquisition are recognized as the main causes of the residual departures of the experimental curves from the expected behaviour in Fig. 4 . As a general remark applying to both classes of studied states, we note that our numerical models depend strongly on the detection efficiencies (see Supplementary Figs 4 and 5 ). In this sense, the more pronounced discrepancies in Figs 3 and 4 , such as that in the P (0, 2) terms, may be due to noise affecting our estimation of these parameters. More details on the theoretical model for both the SSPS and the TMSS can be found in Supplementary Notes 1 and 2 . Generalized Bell inequalities for WFH detection Correlations such as those revealed in our experiment need to be understood in relation to canonical criteria for non-classicality, for instance the violation of a Bell inequality, to assess their role as possible quantum resources [30] . The ability to access and discriminate higher photon numbers leads us to refer to generalized, higher-dimensional Bell inequalities [31] , which we study theoretically in the context of our experiment with a TMSS. To this end, let us consider the scenario depicted in Fig. 5 . Each mode of a TMSS is analysed by means of a WFH detector; here all four outputs are monitored by perfect PNRDs. We take into account the Fock layers that lead to the detection of M photons on each side: the detected photons are split among the two output ports of the polarizing beam splitters (PBSs) (that is, the photons are either transmitted or reflected) according to the convention indicated in Fig. 5a . Specifically, we consider measurements with D = M +1 possible results, distinguished according to the number of photons Γ detected on the transmitted arm of each PBS. We are thus interested in the probabilities associated with joint detection events comprising outcomes (on each output arm, on both sides) differing by ε (the outcomes being taken modulo D ). { α , α ′} and { β , β ′} denote the LO settings on side A and side B, respectively. 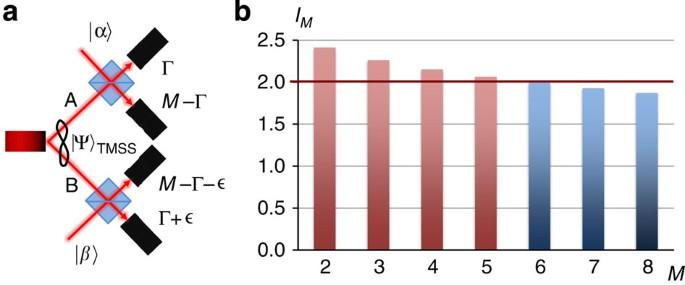Figure 5: Generalized Bell inequalities with WFH. (a) In the ideal case, the two modes of a TMSS are interfered with two weak LOs; PNRDs monitor all four outputs. We fix the number of detected photons toMon each side and label the various detection events recorded by the PNRDs according to how theMparticles distribute themselves on the two output modes: Γ,M−Γ, Γ+ε andM−Γ−ε (b) The plot shows the values taken by the quantityIM(see equation (5)) when the number of detected photonsMon each side varies between two and eight. The bound forIMpredicted by local realism is two for all values ofM, hence we see that no violation of a generalized Bell inequality is possible beyondM=5. The relevant probabilities are combined into the expression Figure 5: Generalized Bell inequalities with WFH. ( a ) In the ideal case, the two modes of a TMSS are interfered with two weak LOs; PNRDs monitor all four outputs. We fix the number of detected photons to M on each side and label the various detection events recorded by the PNRDs according to how the M particles distribute themselves on the two output modes: Γ, M −Γ, Γ+ε and M −Γ−ε ( b ) The plot shows the values taken by the quantity I M (see equation (5)) when the number of detected photons M on each side varies between two and eight. The bound for I M predicted by local realism is two for all values of M , hence we see that no violation of a generalized Bell inequality is possible beyond M =5. Full size image where the local realistic bound is | I M |≤2 (ref. 31 ). We note that the case M =1 corresponds to the standard CHSH inequality that was experimentally tested in ref. 17 . Additional details on how to compute I M for the specific layout that we consider are provided in Supplementary Note 3 , Supplementary Figs 6 and 7 . We run a numerical search for values of M ranging from 2 to 8 to find the set of parameters { λ , α , α ′, β , β ′} that determine the highest violation of these generalized Bell inequalities. Our results are shown in Fig. 5b : no violation of equation (5) is found beyond M =5. This behaviour comes from the fact that the maximal violation of equation (5) (that is, the attainment of the maximum value allowed by quantum mechanics) relies on a particular structure for the entangled state [32] . Notably, a TMSS is specified solely by the squeezing parameter λ : this means that there are not enough degrees of freedom to tune to obtain the required form for the input state. This restriction becomes more severe as the dimensionality of the system increases, to the point that no violation of local realism can be inferred despite the use of an entangled resource such as a TMSS. Hence the decrease in the violation stems from the Gaussian character of the TMSS, which fixes the functional shape of the oscillation curves simultaneously for all Fock layers. We have shown how WFH can be used to deconstruct phase-dependent measurements on two-mode entangled states into their constituent Fock layers. The ability to operate devices at the interface of wave and particle regimes opens up new possibilities for quantum information processing [33] . Thus, our work provides a new insight on such resources within the broader investigations on hybrid continuous/discrete-variable coding [34] , [35] , [36] , [37] , [38] . As a complement, we have also studied the theory of the violation of generalized Bell inequalities using an ideal WFH setup. These tests shed light on how the transition from non-Gaussian to Gaussian measurements occurs. Such transition is achieved in the context of WFH detection as an increase in the LO strength. In fact, this study may also be interpreted in the more general framework of Gaussian versus non-Gaussian measurements, where it is well-known that the outcomes of a Gaussian measurement on a Gaussian quantum state can be explained by a local realistic model. For this reason, strong-field homodyne detection on a TMSS cannot be used to violate a Bell inequality [39] , [40] . On the other hand, weak-field homodyne is an example of non-Gaussian measurement, as attested by its Wigner function. Consequently, we expect that the outcomes of WFH detection on an entangled Gaussian state cannot be described by a local realistic model [17] , [41] , [42] ; however, this breaks for moderately high photon numbers. On the experimental side, further developments for the observation of the violation of higher-dimensional Bell inequalities demand detectors with higher quantum efficiency [43] . These are not only necessary for achieving significant counting statistics, but also to prevent one Fock layer to be affected from higher-order contributions. Encouraging results have been obtained in this direction with cryogenic detectors. Source of quantum states A pulsed Ti:Sapphire laser (repetition rate 256 kHz, central wavelength λ IR =830 nm and bandwidth Δ λ IR ≅ 30 nm) is doubled in a nonlinear crystal (β-barium borate). The second-harmonic beam ( λ UV =415 nm) pumps a type-II parametric downconversion process in a nonlinear crystal (potassium dihydrogen phosphate) to produce a two-mode vacuum-squeezed state. The source is designed to generate spectrally uncorrelated modes based on group velocity mismatch inside the birefringent medium [27] . Daughter photons have orthogonal polarizations and different spectral widths (Δ λ V ≅ 12 nm, Δ λ H ≅ 6 nm). The same source generates the SSPS and the TMSS depending on the ultraviolet pump beam brightness. WFH detection The detection system that we adopt in our experiment is realized with a collinear geometry to ensure passive phase stability. Each mode in equations (1) and (3) is superposed with a LO of orthogonal polarization at a PBS. This delivers a common spatial mode at the output but orthogonal polarizations for the signal to be probed and the weak coherent beam. Interference is then realized by a half-wave plate and an additional PBS. The relative phase between the horizontal and vertical polarizations can be adjusted by means of a geometric phase rotator (GPR—see Fig. 1b ), which is composed of a quarter-wave plate (QWP), a half-wave plate and a second QWP. The axis of the first QWP is set to 45° to transform the input linear polarizations into circular ones. The rotation of the HWP by an angle φ /4 results in a phase shift equal to φ between left- and right-circular polarizations. The initial linear polarizations are then recovered by setting the second QWP to 45°. The successful calibration of the full device relies on the characterization of each element (including the PBS), particularly of the QWPs. When the GPR is correctly calibrated power fluctuations around 3% are recorded, while imperfections in the calibration of one of its constituents can lead to fluctuations in power above 10% (see Supplementary Fig. 2 ). Finally, the output state is analysed with a TMD: this consists of two fibre-based cascaded Mach–Zehnder interferometers that split the incoming state over two spatial modes and four distinct time bins. Time-resolved clicks from avalanche photodiodes monitoring the two transmitted modes are thus registered. Active phase stabilization To actively lock the phase set by the GPRs, we use an ancillary laser beam (from a continuous-wave HeNe laser, λ ′=633 nm), which back-propagates through the interferometer. The classical interference pattern that we obtain when the ancillary beam reproduces correctly the signal and LO optical paths constitutes the signal recorded by a photodiode connected to a PID device (SRS SIM960 Analog PID Controller). How to cite this article: Donati, G. et al. Observing optical coherence across Fock layers with weak-field homodyne detectors. Nat. Commun. 5:5584 doi: 10.1038/ncomms6584 (2014).